Fluorocarbon adsorption in hierarchical porous frameworks Metal-organic frameworks comprise an important class of solid-state materials and have potential for many emerging applications such as energy storage, separation, catalysis and bio-medical. Here we report the adsorption behaviour of a series of fluorocarbon derivatives on a set of microporous and hierarchical mesoporous frameworks. The microporous frameworks show a saturation uptake capacity for dichlorodifluoromethane of >4 mmol g −1 at a very low relative saturation pressure ( P / P o ) of 0.02. In contrast, the mesoporous framework shows an exceptionally high uptake capacity reaching >14 mmol g −1 at P / P o of 0.4. Adsorption affinity in terms of mass loading and isosteric heats of adsorption is found to generally correlate with the polarizability and boiling point of the refrigerant, with dichlorodifluoromethane >chlorodifluoromethane >chlorotrifluoromethane >tetrafluoromethane >methane. These results suggest the possibility of exploiting these sorbents for separation of azeotropic mixtures of fluorocarbons and use in eco-friendly fluorocarbon-based adsorption cooling. Fluorocarbon derivatives are of great practical and industrial interest because of their usefulness in many applications, including fluoropolymers, refrigerants, propellants, solvents, anaesthetics and surfactants, to name just a few. Fluorocarbons also have important environmental significance because of their long lifetime and high ozone depletion and global warming potential. Understanding the adsorption behaviour of fluorocarbons is of fundamental importance in specific applications such as separating mixtures [1] , [2] , [3] , developing thermally driven cooling devices [4] , etching dielectrics for integrated circuits and wastewater cleanup [5] . Motivation for the work described in this paper stems from our group’s research toward developing new adsorption cooling devices using high-performance metal-organic framework (MOF) sorbents and fluorocarbon refrigerants [6] . Sorbents examined for fluorocarbon-based adsorption chillers have thus far been limited to activated carbon [7] , [8] and zeolites [9] . Although the literature on gas adsorption in MOFs is very extensive [10] , [11] , [12] , [13] , [14] , [15] , [16] , [17] , [18] , [19] , fluorocarbon adsorption has been limited to zeolites and activated carbons [7] , [8] , [9] . The adsorption behaviour of the MOFs with high capacity at very low vapor pressures suggests MOFs can, in principle, be used in fluorocarbon-based adsorption heat pumps, separation of fluorocarbons from azeotrope mixture, removal of environmentally hazardous gases from atmosphere. Hence, this paper represents the systematic study of the interaction of fluorocarbon refrigerants with MOFs and the proof of concept for separation of fluorocarbons using crystalline MOFs. MOF selection Two classes of MOFs were selected for the adsorption study: microporous MDOBDC (M=Ni and Co; DOBDC=2,5-dioxido-1,4-benzenedicarboxylate) with a high density of open metal sites [20] , and MIL-100(Fe) [21] and MIL-101 (ref. 22 ) with a hierarchical pore structure. MDOBDC has a uniform, 1.1-nm cylindrical pore ( Fig. 1a ), while MIL-101 consists of two types of mesoporous cages (~25–29 Å) connected through microporous pentagonal (~11.7 Å) and hexagonal windows (~16 Å). Similarly, MIL-100(Fe) consists of mesoporous cages (24–30 Å) connected through pentagonal and hexagonal windows 5–8 Å in size ( Fig. 1b ). In this regard, several groups have shown these two classes of MOFs have extremely high adsorption capacity at room temperature compare with any other MOFs reported thus far [20] , [21] , [22] . For example, water adsorption capacity in MIL-101 is the highest to date and completely reversible up to 100 cycles [23] . Whereas MDOBDC (M=Ni, Mg, Co) MOFs shown to have high CO 2 uptake capacity at P/P0=0.14bar [24] . This was explained by the presence of higher density of open metal cites in a nanopore. Apart from these, MDOBDC- and MIL-101-based MOFs are easier to synthesize compare with other high surface area MOFs. Therefore, selecting DOBDC- and MIL-based MOFs allows investigation of the effects of pore morphology on refrigerant adsorption and selectivity. Similarly, sorption of the commercially available refrigerants shown in Fig. 1c was measured on each MOF. Before the adsorption experiments, all of the MOFs were synthesized and characterized using powder X-ray diffraction and Brunauer–Emmett–Teller surface area analysis ( Supplementary Figs 1 and 2 ). 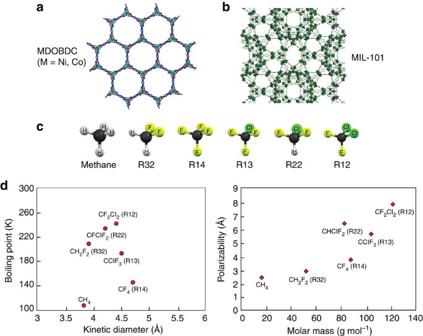Figure 1: Types of MOFs and fluorocarbons investigated. Crystal structures of NiDOBDC (a), MIL-101 (b) and fluorocarbons (c). Physical parameters of fluorocarbons including boiling point, kinetic diameter and polarizability (d). Notice the increase in polarizability and boiling points from methane to dichlorodifluoromethane (R12). Figure 1: Types of MOFs and fluorocarbons investigated. Crystal structures of NiDOBDC ( a ), MIL-101 ( b ) and fluorocarbons ( c ). Physical parameters of fluorocarbons including boiling point, kinetic diameter and polarizability ( d ). Notice the increase in polarizability and boiling points from methane to dichlorodifluoromethane (R12). Full size image Fluorocarbon adsorption Adsorption/desorption of R12 (Dichlorodifluoromethane, CCl 2 F 2 ) on MDOBDC, MIL-101, and MIL-100(Fe) at 298 K are shown in Fig. 2a . All adsorbents display a typical type-I adsorption isotherm at room temperature; however, uptake of R12 by NiDOBDC and CoDOBDC are extremely high even at very low relative vapor pressures (~60 mass%, 5 mmol g −1 ). The saturation capacity of R12 in MIL-101 is 180 mass% (15 mmol g −1 ) at 4 bar ( P / P o =0.6), but reaches 90% of its total capacity at 2 bar. The saturation capacity of MIL-101 is twice that of MDOBDC and MIL-100(Fe) (80 mass%, 6.7 mmol g −1 ). At low pressure ( P / P o=0.01), both DOBDC MOFs adsorb (4.58 mmol g −1 ) more than twice the capacity of MIL-101 (<2 mmol g −1 ) and reach saturation at P / P o=0.05 ( Supplementary Fig. 3 ). These findings are consistent with MOFs containing a high density of open metal sites playing a crucial role in sorbate–sorbent interactions and are similar to the observations reported by others [24] , [25] , [26] , [27] , [28] . Desorption profiles indicate no obvious hysteresis for R12, indicating moderate sorbate–sorbent interactions ( Supplementary Figs 3–5 ). 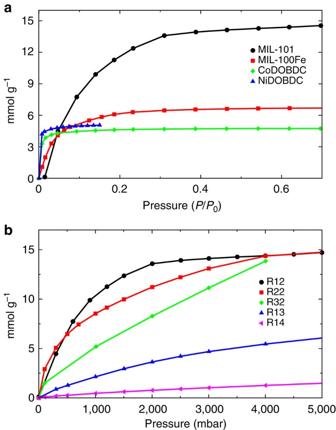Figure 2: Fluorocarbon adsorption in MOFs. Adsorption isotherms of R12 at 298 K in MDOBDC (M=Ni, Co), MIL-100(Fe) and MIL-101 (a). Sorption profiles of various refrigerants in MIL-101 at 298 K (b). Figure 2: Fluorocarbon adsorption in MOFs. Adsorption isotherms of R12 at 298 K in MDOBDC (M=Ni, Co), MIL-100(Fe) and MIL-101 ( a ). Sorption profiles of various refrigerants in MIL-101 at 298 K ( b ). Full size image The adsorption capacity of all the refrigerants in MIL-101 at room temperature is shown in Fig. 2b . As expected, the adsorption capacity of R12 is higher than in closely related analogues at 2 bar pressure; the uptake values are 14 mmol g −1 of R12 (180 mass%), 11 mmol g −1 (120 mass%) of R22(Chlorodifluoromethane, CHClF 2 ), 4 mmol g −1 (80 wt%) of R13 (Chlorotrifluoromethane, CClF 3 ), 8 mmol g −1 of R32(Difluoromethane, CH 2 F 2 ) and <1 mmol g −1 (20 mass%) of R14 (Tetrafluoromethane, CF 4 ), respectively. At low pressure (<500 mbar), the adsorption of R22 in MIL-101 is significantly higher than that of R12, R13 and R14. Grand Canonical Monte Carlo (GCMC) simulations were performed to confirm the uptake capacities obtained experimentally for MIL-101 and NiDOBDC ( Supplementary Figs 6 and 7 ). The simulation snapshots suggest that at low pressure, R12 preferentially occupies Ni 2+ sites in NiDOBDC ( Supplementary Fig. 8 ). Similarly in MIL-101, R12 preferentially adsorbs in small pockets because of the efficient overlap between refrigerant molecules and the smaller cage, but as the pressure increases, both R12 and R22 fill the rest of the cage structure leading to similar loadings at saturation ( Supplementary Figs 9,10 ). Isosteric heats of adsorption Qst at a constant loading were calculated from fitting the adsorption isotherms at different temperatures (288, 298 and 308 K) to a Clausius–Clapeyron equation ( Supplementary Fig. 11 ). Higher enthalpies of adsorption at lower loadings were observed and constantly decrease as refrigerant loading increases ( Supplementary Fig. 12 ). Adsorption enthalpy of R22 (34.6 kJ mol −1 ) is considerably higher in magnitude compared with R12, R13, R14 and R32 (refs 25 , 26 ). The Qst values are higher than the standard enthalpy of vaporization for R12, R22 (20 and 28.2 kJ mol −1 ) and similar to the Qst for MOFs with open metal sites such as MDOBDC (CO 2 as sorbate) [14] , [29] , [30] . Molecular simulation and solid-state NMR To better understand how the orientation and distribution of R12 inside the MIL-101, we computed radial distribution functions (RDFs) by performing molecular dynamics simulations. The computed RDFs are shown in Fig. 3a–c , where the distance between the carbon atom of R12 (C R12 ) and carbon atoms within the phenyl ring of MIL-101 (C phenyl ) and Cr 3+ . Similarly, RDF plots were generated for chlorine and fluorine atoms of R12 (Cl R12 and F R12 ) with respect to Cr 3+ in MIL-101. The RDF distance plot with respect to MIL-101 clearly shows that R12 is closer to Cr 3+ than the phenyl group, and F R12 is closer to Cr 3+ than the Cl R12 , indicating that in R12, the F R12 faces toward the Cr 3+ sites because of the favourable C–F···M + interactions between the fluorine of R12 and Cr 3+ sites ( Fig. 3b ). The calculated bond length and angle between C–F R12 ···Cr 3+ MIL-101 was 2.27 Å and 110 ° with a slight elongation of C–F R12 bond length (1.39 Å) caused by the weak attractive forces. These C–F···M + interactions are consistent with previous crystallographic and NMR experiments on metal complexes of fluorine-containing cage compounds and suggest short C−F···M + distances and elongation of C−F bonds in the crystal structure [31] . 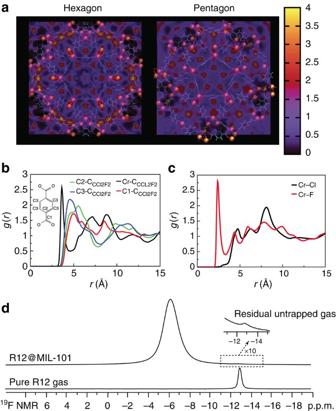Figure 3: Modelling and solid-state19F NMR. The RDF computed from the molecular dynamics simulations of loading R12 in MIL-101 at 2,000 mbar and 298 K. Hexagons of MIL-101 are large enough that they contain two solvation shells of R12 molecules, while triangular shapes are the perfect size to accommodate one R12 molecule (a). RDF between CR12and different atoms of MIL-101 (b). RDF between ClR12and FR12and the Cr3+MIL-101(c).19F MAS NMR spectrum of R12 in MIL-101. Notice the downfield shift of R12 in the pores (d). Figure 3: Modelling and solid-state 19 F NMR. The RDF computed from the molecular dynamics simulations of loading R12 in MIL-101 at 2,000 mbar and 298 K. Hexagons of MIL-101 are large enough that they contain two solvation shells of R12 molecules, while triangular shapes are the perfect size to accommodate one R12 molecule ( a ). RDF between C R12 and different atoms of MIL-101 ( b ). RDF between Cl R12 and F R12 and the Cr 3+ MIL-101 ( c ). 19 F MAS NMR spectrum of R12 in MIL-101. Notice the downfield shift of R12 in the pores ( d ). Full size image Solid-state 19 F magic angle spinning (MAS) NMR of MIL-101-containing R12 shows the resonance of the stored R12 as a sharp signal around −6 p.p.m. compared with free gas at −12.8 p.p.m. ( Fig. 3d ). Similarly, the sample containing R22 shows a single resonance at −67.5 p.p.m. compared with the gas phase R22, which appears at −77.5 p.p.m. ( Supplementary Fig. 13 ). These exceptional shifts are robust experimental evidence of gas trapped within the pores of the MOF. The observed low field shift (towards higher p.p.m.) is caused by strong interaction between the loaded gas molecules and paramagnetic chromium metal centre in the host lattice. In addition, the single resonance 19 F MAS NMR peak for R12 and R22 indicate that all of the fluorines are preferentially aligned toward Cr 3+ through electrostatic interactions, which was clearly observed in our modelling studies. Because of the strong binding energies of refrigerant molecules with MIL-101, we calculated the density of R12 in the pores at STP to be 1.12 g cm −3 , or 225 times its vapor density. Similarly, the calculated densities of other refrigerants in MIL-101 at STP are 0.82 (R22), 0.11 (R14) and 0.51 g cm −3 (R13), respectively. Fluorocarbon separation To further demonstrate the applicability of MIL-101 for separation of fluorocarbons, experiments were conducted using a custom built breakthrough reactor coupled with residual gas analyzer (RGA; Supplementary Fig. 14 ) [32] , [33] . Around 130 mg of MIL-101 was packed in a column and the sample was activated at 200 °C by flowing Helium overnight. The column was cooled down to room temperature and introduced a mixture of 90% He, 2% R22 and 8% of R12 with a flow rate of 0.25 ml min −1 at a total pressure of 10 bar. The Helium broke through the column immediately after injection (<1 min) indicating MIL-101 does not have any selectivity towards Helium gas. After 30 min of injection, R22 broke through the column followed by R12 at 50 min, indicating preferential adsorption and selectivity towards R12 over R22 by MIL-101 ( Fig. 4 , Supplementary Fig. 15 ). The experimental breakthrough measurements are in line with experimental pure gas isotherms where MIL-101 shows R12 has higher adsorption capacity than R22 at room temperature and pressure of 800 mbar. Complementary to experimental breakthrough, using the pure component adsorption isotherms, we carried out simulations of the breakthrough of an equimolar four-component R12/R13/R14/R22 mixture in a fixed bed packed with MIL-101 ( Supplementary Figs 16–22 and Supplementary Methods ); the simulation methodology is outlined elsewhere [34] , [35] . Fig. 5a demonstrates that MIL-101 effectively separates the mixture into individual fractions. The separation of a mixture of R12 and R22 with the azeotropic composition is also feasible, as demonstrated by the breakthrough calculations depicted in Fig. 5b . 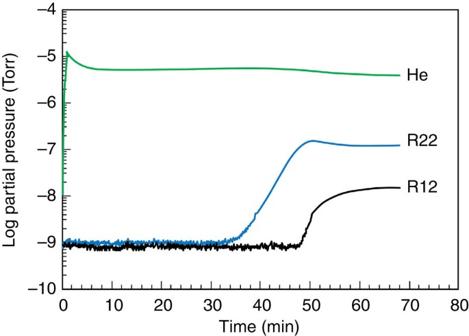Figure 4: Fluorocarbon separation. Experimental breakthrough of adsorption bed packed with MIL-101, a mixture of 90% He, 2% R22 and 8% of R12 fed through the column with a flow rate of 0.25 ml min−1. Figure 4: Fluorocarbon separation. Experimental breakthrough of adsorption bed packed with MIL-101, a mixture of 90% He, 2% R22 and 8% of R12 fed through the column with a flow rate of 0.25 ml min −1 . 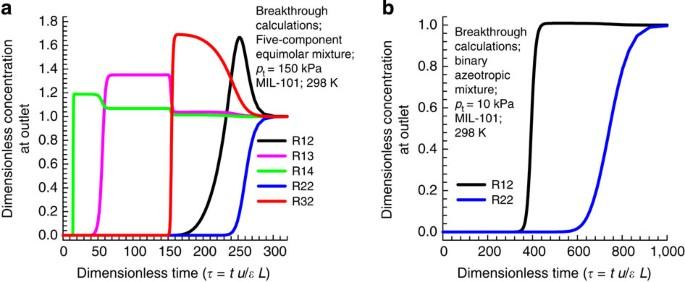Figure 5: Simulated breakthrough experiments. Breakthrough characteristics of an adsorber packed with MIL-101. R22 separates from a feed of equimolar R12/R22/R13/R14/R32 mixture (a); azeotrope mixture consists of 98% R12 and 2% R22 (b). Full size image Figure 5: Simulated breakthrough experiments. Breakthrough characteristics of an adsorber packed with MIL-101. R22 separates from a feed of equimolar R12/R22/R13/R14/R32 mixture ( a ); azeotrope mixture consists of 98% R12 and 2% R22 ( b ). Full size image Two classes of porous MOF containing high density of open metal sites with uniform cylindrical pore structure (MDOBDC) and mesoporous cages connected through microporous windows (MIL-101) were investigated for fluorocarbon adsorption and separation. The microporous MDOBDC MOFs showed a saturation uptake capacity for fluorocarbons of >4 mmol g −1 at a very low relative saturation pressure ( P / P o ) of 0.02. In contrast, the mesoporous framework showed an exceptionally high uptake capacity reaching >14 mmol g −1 at P / P o of 0.4. Our results are in consistent with MOFs containing a high density of open metal sites playing a crucial role in sorbate–sorbent interaction. Further adsorption affinity generally declines in accordance with decreasing polarizability of the refrigerant ( Fig. 1 ) reflecting the strong influence of non-covalent interactions with the coordinatively unsaturated metal centres in the MOF. Similarly, we can correlate the adsorption of a gas to its boiling point. The higher boiling point roughly means stronger gas···gas interactions. Hence, more likely for higher boiling point gas will have stronger host···gas interactions. This trend was clearly observed with gases CO 2 , N 2 , O 2 , H 2 and CH 4 , where CO 2 will adsorb onto host surface preferentially over other gases because of higher boiling point and stronger forces between MOF and CO 2 compare with other gas molecules. Similar trend was observed with fluorocarbons and MOFs discussed here, the higher refrigerant boiling point has high adsorption capacity and Q st as discussed above. In addition, a close inspection of Q st data indicates that R22 has slightly higher enthalpy of adsorption at lower loadings than R12, though R22 has lower polarizability and boiling point. This could be explained by the presence of three electron-withdrawing groups in R22; these groups make the available hydrogen very acidic, and R22 is smaller in kinetic diameter and more polar than R12. The dipole moments are 1.42 (R22), 1.98 (R32) and 0.61 (R12) Debye units, respectively. According to the hydrogen bond acid–base theory, the acidic protons in R22 are a good hydrogen bond donor. As a result, R22 forms stronger C–H···π/C–H···O interactions with the phenyl groups in MIL-101, whereas R12 interactions are purely based on polarizability. This observation is further supported by density functional theory calculations and GCMC simulation snapshots where R22 molecules are oriented towards the phenyl groups of MIL-101 at low pressures ( Supplementary Figs 9 and 10 , Supplementary Tables 1 and 2 ). Due to the difference in adsorption affinity of fluorocarbons, MIL-101 effectively separates the mixture into individual fractions as reflected in the simulation and experimental breakthrough measurements. These results demonstrate the proof of concept for separation of fluorocarbons using few selected MOFs, however additional work on related MOFs (MOF-210, NU-100, PCN-14, Bio-MOF-100, UMCM-1, NOTT-100) [29] , [36] , [37] , [38] , [39] , [40] and covalent organic frameworks [41] is under investigation to further improve the adsorption capacity and selectivity of fluorocarbons. In conclusion, the discovery of exceptionally high capacity and reversible adsorption of fluorocarbon refrigerants in porous crystalline MOFs at room temperature suggests the possibility of exploiting these sorbent materials for eco-friendly adsorption cooling applications and separation of mixtures of chlorofluorocarbons from hydrochlorofluorocarbons and hydrofluorocarbons. The adsorption behaviour of the MDOBDC MOFs with high capacity at very low vapor pressures suggests strong potential for application in refrigeration or even cryogenic solid-state cooling devices. General procedures and protocols All the starting materials including solvents used in the synthesis were purchased from Aldrich Chemicals and were used without further purification. The powder X-ray diffraction measurements were performed on Bruker AXS D 8 Discover powder diffractometer at 45 kV, 200 mA for Cu Kα ( λ =1.5406 Å) and the purity and homogeneity of the bulk samples were determined by comparison of the simulated powder patterns which were calculated using Mercury 3.1. All thermogravimetric analysis experiments were performed using Netzsch TG209 F1 under a N 2 atmosphere from 25 to 500 °C at a rate of 5 °C min −1 . Synthesis of MIL-101 In brief, 1 mmol of 1,4-benzenedicarboxylic acid (H 2 BDC, 166 mg) was added to tetramethylammonium hydroxide solution (5 ml, 0.05 mol l −1 ) and stirred at room temperature for 10 min. To this solution, 1 mmol of chromium (III) nitrate nonahydrate (Cr(NO 3 ) 3 ·9H 2 O; 400 mg) was added and maintained at pH 6.0–6.5. The reaction mixture was stirred for 20 min and then transferred into a 23-ml Teflon-lined autoclave and heated for 24 h at a temperature of 180 °C. After slowly cooling to room temperature, the green powder was collected by repeated centrifugation and thoroughly washed with distilled water, methanol and acetone. Synthesis of MIL-100(Fe) A solution containing Fe-powder (10 mmol, 555 g), 1,3,5-benzene tricarboxylic acid (H 3 BTC) (6.5 mmol, 1.375 g), hydrofluoric acid (0.4 ml, nitric acid (0.76 ml) and deionized water (50 ml) was placed in a 125-ml Teflon-liner. The Teflon-liner was placed in an autoclave and heated to 150 °C. After 6 days, the autoclave was cooled to room temperature within 24 h. The reaction mixture was filtered, and the solid light-orange product was heated in water for 3 h at 80 °C. The product was filtered and air-dried at room temperature. Synthesis of MDOBDC (M=Ni, Co) To a solid mixture of 2,5-dihydroxyterephthalic acid (0.12 mmol, 1 equival.) and corresponding metal nitrates (Ni or Co, 0.40 mmol, 3.33 equival.) were added to a 1:1:1 (v/v/v) mixture of DMF–ethanol–water in a Teflon jar contained in a stainless steel autoclave with Teflon screw-cap. The reaction mixture was mixed thoroughly followed by ultrasonication for 15 min to get a homogeneous clear solution. The reaction solution was then placed in an oven at 100 °C for 24 h and then slowly cooled to room temperature. The mother liquor was decanted from the yellow microcrystalline material and thus obtained yellowish microcrystalline compound was washed several times with methanol followed by soaking in fresh methanol for 72 h while replacing fresh methanol for every 24 h. The solvent was removed under vacuum at 250 °C over 10 h to activate the material. Fluorocarbon adsorption and IAST calculations The adsorption experiments using fluorocarbons were carried out using Intelligent Gravimetric Analyzer from Hiden Instruments. The methanol exchanged MIL-101 was activated at 250 °C (5 °C min −1 ) under vacuum for 12 h. After activation, the dry mass of the adsorbent was corrected and the experimental temperatures were maintained thought out each sorption experiment using a water bath. A specific amount of fluorocarbon gas introduced into the sample chamber and the pressure was maintained at each set point for about 20 min until equilibrium is established. The mass uptake was measured as a function of pressure until equilibrium was established, at which point the pressure was increased to the next set pressure value and the subsequent uptake was measured until equilibrium was re-established. The experimentally measured loadings of R12, R13, R14, R22 and R32 in MIL-101 were fitted with the dual-site Langmuir–Freundlich model. The fits are excellent over the entire range of pressures ( Supplementary Fig. 16 ). To determine the potential of MIL-101 to separate mixtures containing R12, R13, R14, R22 and R32, we calculated the component loadings in MIL-101 in equilibrium with an equimolar five-component mixture in the gas phase. The calculations of the Ideal Adsorbed Solution Theory of Myers and Prausnitz [42] for the component loadings for a range of total bulk gas phase pressures ( Supplementary Methods ). Solid-state 19F NMR 19 F NMR measurements were made using a Varian 850 Inova magnet ( B 0 =19.97T and 19 F Larmor frequency of 799.54 MHz) with MAS at 15 kHz using 3.2-mm zirconia rotors. All measurements were done immediately after gas loading in MOF samples to avoid any desorption caused by prolonged exposure to atmospheric pressure. Chemical shifts were referenced to aqueous sodium trifluoroacetate samples ( δ iso =−76.5 p.p.m. with respect to CFCl 3 δ iso =0 p.p.m.) at spinning speeds of 10 kHz. The estimated uncertainty in chemical shifts was 0.05 p.p.m., and was determined through calibration using the sodium trifluoroacetate reference sample. GCMC simulations GCMC simulations were carried out using the MUSIC programme [43] . The simulation box consisted of a unit cell of MIL-101 with periodic boundary conditions used in all three dimensions. During the simulations, both MIL-101 framework and the fluorocarbon molecules are kept rigid. Intermolecular interactions between the framework and fluorocarbon molecules were described by Lennard–Jones and Electrostatic interactions and are evaluated using standard Wolf method. The force-field parameters for MIL-101 was used from the density-functional theory studies [44] , [45] . Force-field parameters were developed for R12 by carrying out a series of molecular dynamics simulations until the experimental density and heat of enthalpy were reproduced ( Supplementary Table 3 ). For each simulation run, the chemical potential ( μ ), volume ( V ), and temperature ( T ) were fixed (grand canonical ensemble, μVT ). The chemical potential of R12 was calculated using the ideal gas law. GCMC simulations were performed with four types of moves: (1) molecular displacement, (2) molecular rotation, (3) insertion of a molecule with random orientation into a random position in the system and (4) deletion of a randomly chosen molecule from the system. At each pressure and temperature points, we performed 10 7 trial moves for GCMC simulations. Density functional theory calculations are performed to compute the binding energies for organic linker and the guest molecules at different orientations. NWCHEM computational package is used with M06 functional and 6-31G** basis set. For the case of R12 geometry, optimization is carried and energies are computed for two conformations with chlorine and fluorine oriented in the perpendicular to plane of aromatic ring. Similarly, for the case of R22, we explored three conformations with hydrogen, chlorine, fluorine perpendicular to the plane of the aromatic ring. Experimental breakthrough Breakthrough measurements were conducted by packing 130 mg of MIL-101 in a 6.35-cm long and 0.5-cm diameter column. The sample was activated at 200 °C with flowing helium overnight. Pressurization of the 0.25" (6.35 mm) diameter column packed with MOF was accomplished with a syringe pump (Teledyne ISCO) directly connected to the system through a series of 0.07 mm (ID) segments of tubing (PEEK) and valves. System pressure was maintained by coordinated adjustments to the syringe pump flow rate and the needle metering valve (Tescom). An inline pressure transducer was used to verify column pressure. The column was cooled to room temperature and a mixture of 90% He, 2% R22 and 8% of R12 was introduced with a flow rate of 0.25 ml min −1 at a total pressure of 10 bar. Effluent gas chemistry was tracked with a Stanford Research residual gas analyzer (RGA). Masses (a.m.u.) corresponding to He (4), R12 (103) and R22 (51) were monitored throughout the experiments. The flow rate through the needle metering valve created a sampling pressure of 1.0 to 3.0 × 10 −4 Torr in the RGA and was maintained throughout the experiments. Indications of R12 and R22 breaking through the column were indicated by an increase in the pressure for masses 103 and 51 respectively. Similarly, simulated breakthrough experiments were conducted using five-component and azeotropic mixure using MIL-101 and details were provided in Supplementary Figs 16–22 and Supplementary Table 4 . How to cite this article : Motkuri, R. K. et al. Fluorocarbon adsorption in hierarchical porous frameworks. Nat. Commun. 5:4368 doi: 10.1038/ncomms5368 (2014).